Lymphocytes can self-steer passively with wind vane uropods A wide variety of cells migrate directionally in response to chemical or mechanical cues, however the mechanisms involved in cue detection and translation into directed movement are debatable. Here we investigate a model of lymphocyte migration on the inner surface of blood vessels. Cells orient their migration against fluid flow, suggesting the existence of an adaptive mechano-tranduction mechanism. We find that flow detection may not require molecular mechano-sensors of shear stress, and detection of flow direction can be achieved by the orientation in the flow of the non-adherent cell rear, the uropod. Uropods act as microscopic wind vanes that can transmit detection of flow direction into cell steering via the on-going machinery of polarity maintenance, without the need for novel internal guidance signalling triggered by flow. Contrary to chemotaxis, which implies active regulation of cue-dependent signalling, upstream flow mechanotaxis of lymphocytes may only rely on a passive self-steering mechanism. Cell migration plays an essential role in the living world, from nutrient searching in mono-cellular organisms to morphogenesis, tissue repair and immune cells patrolling in multicellular organisms. To perform such complex tasks efficiently, cells are frequently guided towards targeted locations by various external cues such as soluble chemicals (chemotaxis), surface-bound chemicals (haptotaxis) or mechanical stimuli such as substrate stiffness, cell deformation or hydrodynamic stress (mechanotaxis). Guiding mechanisms have long been studied and yet many aspects of these sophisticated processes remain unexplained. We are interested here in the recently observed phenomenon of leukocyte guidance by a hydrodynamic flow. Before extravasation from the blood stream into tissues, circulating leukocytes arrest and crawl with an amoeboid motility [1] on the luminal surface of blood vessels under the influence of an intense shear stress exerted by flowing blood. The role of flow on leukocyte crawling and extravasation remains generally an unsolved question [2] ; however, crawling T lymphocytes were recently reported in vivo [3] and in vitro [4] to orient against the direction of flow and to move upstream similar to salmon in a river. This non-intuitive behaviour is manifestly not a drift of cells pushed by the flow, and we sought here to clarify the origin, role and mechanism of this upstream flow mechanotactic behaviour. Eukaryotic chemotaxis is the most prominent and studied guidance mechanism. Signal detection by cells exposed to a soluble chemical gradient occurs via known molecular sensors (G-protein-coupled receptors) that are specific for various factors. They are usually distributed fairly evenly on the cell surface [5] , [6] and produce a differential outside/inside signalling between the front and rear of cells ( Fig. 1a ). A complex signalling pathway eventually yields a polarized phenotype with biased motility towards the gradient [7] . In comparison, the deciphering of mechanotaxis is much less advanced. Relatively few molecules have been identified as potential mechanical sensors, for instance, the Src kinase substrate p130Cas, which is phosphorylated under an extension force [8] . As adaptive phosphorylation of p130Cas was reported to be involved in the downstream orientation of endothelial cells [9] , one may imagine an active mechanism analogous to chemotaxis for flow mechanotaxis, involving local molecular sensing of external cues and specific internal signalling to reorient migration. Yet, a critical consideration is that while chemical concentration and substrate rigidity in chemotaxis and mechanotaxis, respectively, are gradient signals, the hydrodynamic shear stress in flow mechanotaxis is homogeneous in the plane of cellular displacement. A chemotaxis-analogue scenario with molecular force sensors homogeneously distributed would therefore yield a non-polarized internal signalling and no directional sensing ( Fig. 1b ). A polarized repartition of molecular sensor ( Fig. 1c ) or cell morphology ( Fig. 1d ) could generate a differential rear-front signalling under homogeneous stress. However, the existing polarization axis would be enhanced under flow but would not depend on the direction of flow. Flow mechanotaxis seems, therefore, intrinsically incompatible with a local detection by molecular sensors of force only, which suggests that a structural organization at the supramolecular [9] or cellular level is required. The location and the type of detection involved in the flow-depended migration of T lymphocytes remain therefore unclear. 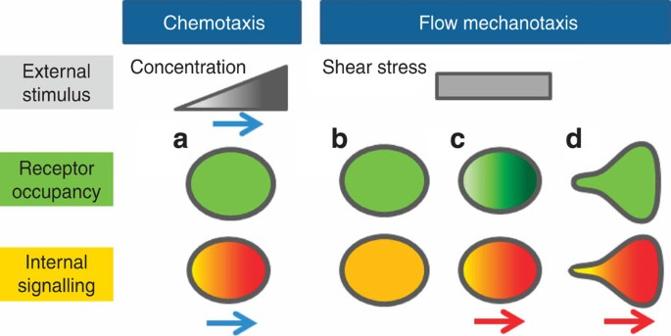Figure 1: From local detection of an external cue to global cellular guiding. Schematic mechanistic pictures for chemotaxis and flow mechanotaxis of the spatial variation of (grey) the external stimuli, (green) the molecular sensor distribution and (orange) the cell internal signalling by molecular sensors. Darker colour represents higher intensities. (a) In chemotaxis, the external cue is a gradient of bulk concentration. Local molecular sensors of concentration evenly distributed5on cells induce internal polarized signalling in line with the direction of the gradient cue (blue arrows). (b–d) In flow mechanotaxis, the external cue (shear stress) is homogeneous in the plane of displacement. In hypothetical models involving local molecular sensors of force, that is, symmetric cell with homogenous (b) and inhomogeneous (c) sensor occupancy, and (d) asymmetric cell with homogeneous sensor occupation, the direction of internal signalling (red arrow) corresponds to a reinforcement of rear-front polarization that is independent of flow direction. Figure 1: From local detection of an external cue to global cellular guiding. Schematic mechanistic pictures for chemotaxis and flow mechanotaxis of the spatial variation of (grey) the external stimuli, (green) the molecular sensor distribution and (orange) the cell internal signalling by molecular sensors. Darker colour represents higher intensities. ( a ) In chemotaxis, the external cue is a gradient of bulk concentration. Local molecular sensors of concentration evenly distributed [5] on cells induce internal polarized signalling in line with the direction of the gradient cue (blue arrows). ( b – d ) In flow mechanotaxis, the external cue (shear stress) is homogeneous in the plane of displacement. In hypothetical models involving local molecular sensors of force, that is, symmetric cell with homogenous ( b ) and inhomogeneous ( c ) sensor occupancy, and ( d ) asymmetric cell with homogeneous sensor occupation, the direction of internal signalling (red arrow) corresponds to a reinforcement of rear-front polarization that is independent of flow direction. Full size image Herein, we analysed the mechanism of T lymphocyte guidance under flow using microfluidic devices to impose changes of flow direction and magnetic beads to exert localized forces on the cell body. We show that detection of flow direction when lymphocytes crawl against the flow is achieved at the organelle level by the cell rear, or uropod, that orients in the flow such as a wind vane. Singularly, upstream migration was not hampered by inhibition of classical guidance signalling pathways, and changes in the direction or intensity of flow did not trigger calcium signalling, which together challenge the relevance of an active guidance mechanism. We show, however, that the maintenance of a single-polarity axis with an aligned lamellipod and uropod can spontaneously induce cells to face the flow when their uropod orients similar to a wind vane. Given the intrinsic polarity of the T cells, this process can be characterized as passive steering since it is built on pre-existing polarity signalling structures that do not need to be induced by the flow or magnetic stimulus. Cells uropods reorient with flow direction similar to a wind vane We used primary human effector T lymphocytes on intercellular adhesion molecule 1 (ICAM-1)-coated glass substrates as a minimal in vitro model system to study crawling orientation under flow ( Fig. 2a ). Without additional chemical or mechanical cue, these cells are polarized, adherent and spontaneously motile. An active lamellipod, which extends in the cell front, is considered to act as the motor of the migration machinery via actin polymerization [10] . The central body is mainly occupied by the nucleus and at the cell rear, the uropod is a characteristic organelle of T lymphocytes whose role in cell migration remains enigmatic [11] . In the absence of flow, crawling cells display a random motion with a velocity ~20 μm min −1 and a persistence length ~50 μm, whereas in a unidirectional flow corresponding to a shear stress of 10 dyn cm −2 , all T lymphocytes orient their migration direction upstream ( Fig. 2b ). The total shear force on the cells (~100 pN at 10 dyn cm −2 ) is known to be negligible as compared with the force developed by the powerful motility machinery in the lamellipod (>1,000 pN; ref. 4 ). This has previously permitted us to explain why cell velocity remains unaffected by flow [4] , but it also supports the idea that migration orientation is a specific adaptation of lymphocytes to the relatively faint hydrodynamic cue. However, it is unknown whether this adaptation is active or passive, or whether it arises from the cell front (lamellipod) or cell rear (uropod). For instance, polarized cells are commonly described as being more sensitive to chemoattractant at the anterior than at the posterior [5] . Recent microfluidics experiments on neutrophil chemotaxis show indeed that a cell engages a turn when its leading edge only is exposed to a 90° change of chemical cue direction [12] . Similarly, we used a microfluidic chamber to expose lymphocytes to a 90° change in flow direction ( Fig. 2c , and Supplementary Movies 1 and 2 ). Initially, crawling cells project lamellipods towards the flow and uropods are elongated in their wake. When flow direction changes, the lamellipods growth keeps its original orientation, whereas most uropods are instantaneously pushed sideways or even aligned by the flow of new direction. This observation strongly suggests that uropods may play a leading role in the adaptation of the migration to flow direction. 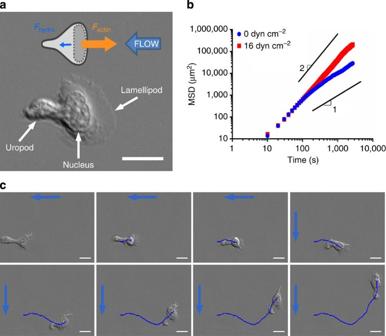Figure 2: Transition from diffusive to directional motility under flow and adaptation to changes of flow direction. (a) Differential interferential contrast image of a lymphocyte crawling on ICAM-1/BSA-coated glass substrate with lamellipod in the front, nucleus in the centre and protruding uropod in the rear. Scale bar, 10 μm. Cartoon represents a crawling lymphocyte under flow with the faint hydrodynamic forceFhydropushing to the left (blue arrow) and the strong internal force due to actin polymerization in the lamellipodFactinpushing to the right (orange arrow). (b) Average mean square displacement (MSD) ofNcelltracked cells as function of time lag in log–log scale. Blue plot: in absence of flow (Ncell=541), the long-term behaviour is almost diffusive (slope 1). Transition between directional and diffusive regime yields a persistence length of 50 μm. Red plot: under a shear stress of 16 dyn cm−2(Ncell=650), the long-term behaviour is almost ballistic (slope 2). (c) Sequence of eight images separated each by 200 s of a crawling lymphocytes under a shear flow of 8 dyn cm−2with a flow (blue arrows) coming first from the right and then from the top (aftert=156 s). Dark blue line traces the track of the cell starting from the first image. Scale bars,10 μm. Figure 2: Transition from diffusive to directional motility under flow and adaptation to changes of flow direction. ( a ) Differential interferential contrast image of a lymphocyte crawling on ICAM-1/BSA-coated glass substrate with lamellipod in the front, nucleus in the centre and protruding uropod in the rear. Scale bar, 10 μm. Cartoon represents a crawling lymphocyte under flow with the faint hydrodynamic force F hydro pushing to the left (blue arrow) and the strong internal force due to actin polymerization in the lamellipod F actin pushing to the right (orange arrow). ( b ) Average mean square displacement (MSD) of N cell tracked cells as function of time lag in log–log scale. Blue plot: in absence of flow ( N cell =541), the long-term behaviour is almost diffusive (slope 1). Transition between directional and diffusive regime yields a persistence length of 50 μm. Red plot: under a shear stress of 16 dyn cm −2 ( N cell =650), the long-term behaviour is almost ballistic (slope 2). ( c ) Sequence of eight images separated each by 200 s of a crawling lymphocytes under a shear flow of 8 dyn cm −2 with a flow (blue arrows) coming first from the right and then from the top (after t =156 s). Dark blue line traces the track of the cell starting from the first image. Scale bars,10 μm. Full size image Uropods can rotate with flow owing to their non-adherence We therefore characterized further the properties of a uropod within its microenvironment. First, the conformation of effector T lymphocytes above the substrates was imaged by confocal microscopy ( Fig. 3a and Supplementary Movie 3 ), which shows that a uropod protrudes typically 10 μm above the surface in absence of flow. Considering the uropod as a vertical cylinder, the force of the flow on the uropod, F u , can be estimated [13] by where z is the height above the surface, μ and ρ are the medium viscosity and density, respectively, R is the radius of the cylinder and V(z) is the fluid velocity at height z . A shear stress σ =10 dyn cm −2 , a uropod length L =10 μm and a radius R =2 μm yield a force F u ≈100 pN. Thus, the hydrodynamic force on the uropod alone is of the same magnitude as that exerted on the whole cell considered as flat, F c = S p σ , with S p ≈100 μm 2 the projected area of individual cells. Indeed fluid velocity at a blood vessel surface is null—according to classical hydrodynamic condition of no-slip at solid surface—and increases linearly away from the surface. The erected uropods expose their extremity to higher fluid velocities that amplifies the force experienced by cell rear for a given flow condition. Second, the footprint of the cell on the substrate was imaged by reflection interference contrast microscopy (RICM; Fig. 3b and Supplementary Movie 4 ). The lamellipod and the central cell body were found to be in close contact with the surface, whereas the uropod was clearly non-adherent. Comparison with total internal reflection fluorescence microscopy (TIRF) images, ( Fig. 3c ) shows that the footprint zone seen in RICM coincides with the presence of integrins. This latter observation is consistent with previous reports of T-cell crawling, showing that adhesion and migration properties are mediated by integrin/ICAM binding and affinity regulation in the front and central body [14] . In contrast, the former observation of non-adherence of the cell rear is surprising relative to existing paradigms on cell motility: for mesenchymatous cells, cell rear is clearly adherent and requires strong actomyosin traction to detach [15] , and for amoeboid cells, actomyosin traction is also reported to be concentrated in uropods [16] . Nevertheless, the non-adherence of lymphocytes uropods is directly relevant for flow-guided migration, as it allows the fast rotation and orientation of uropods with flow in the plane of the substrate, which is similar to a free-rotating wind vane ( Supplementary Note 1 and Supplementary Fig. 1 ). In the end, prominence and most importantly non-adherence make uropods sensitive organelles for detection of flow direction. 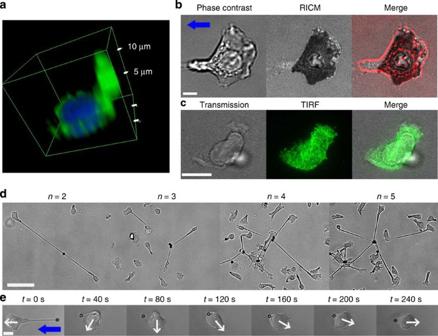Figure 3: Prominent and non-adherent uropods act as wind vanes in the flow and guide cells. (a) Confocal image of a T lymphocyte stained for the membrane (green) and the nucleus (blue) in the absence of flow. (b) T lymphocyte under a shear stress of 8 dyn cm−2in phase contrast mode and in RICM mode. Blue arrow indicates flow direction. Scale bar, 5 μm. (c) Fixed T lymphocyte without flow and in presence of Ab38 against LFA-1 integrins (green) in transmission and TIRF mode. Scale bar, 10 μm. (d) Multiplets of T lymphocytes attached by their uropod to anti-ICAM3-coated beads with number of cellsnper multiplet ranging between 2 and 5. Cells orientation in multiplets is independent of flow direction but multiplets ofncells take quasi-stable star-like conformations with regular angles of 2π/nbetween branches. Scale bar, 50 μm. (e) Image sequence showing the dynamic reorientation of a T lymphocyte in a right to left flow (blue arrow) corresponding to a shear stress of 10 dyn cm−2. Initially, cell faces downstream owing to an attachment of the trailing edge. After the link breaking (t=0 s), it reorients progressively towards the flow. White arrows indicate the instantaneous lamellipod extension direction. Blue arrow indicates flow direction. Scale bar, 10 μm. Figure 3: Prominent and non-adherent uropods act as wind vanes in the flow and guide cells. ( a ) Confocal image of a T lymphocyte stained for the membrane (green) and the nucleus (blue) in the absence of flow. ( b ) T lymphocyte under a shear stress of 8 dyn cm −2 in phase contrast mode and in RICM mode. Blue arrow indicates flow direction. Scale bar, 5 μm. ( c ) Fixed T lymphocyte without flow and in presence of Ab38 against LFA-1 integrins (green) in transmission and TIRF mode. Scale bar, 10 μm. ( d ) Multiplets of T lymphocytes attached by their uropod to anti-ICAM3-coated beads with number of cells n per multiplet ranging between 2 and 5. Cells orientation in multiplets is independent of flow direction but multiplets of n cells take quasi-stable star-like conformations with regular angles of 2 π / n between branches. Scale bar, 50 μm. ( e ) Image sequence showing the dynamic reorientation of a T lymphocyte in a right to left flow (blue arrow) corresponding to a shear stress of 10 dyn cm −2 . Initially, cell faces downstream owing to an attachment of the trailing edge. After the link breaking ( t =0 s), it reorients progressively towards the flow. White arrows indicate the instantaneous lamellipod extension direction. Blue arrow indicates flow direction. Scale bar, 10 μm. Full size image Cell motility direction is opposed to uropod orientation The question remains whether uropods can then transduce their orientation with the flow into a directional cue for migration of cells. We therefore performed a series of experiments to demonstrate that flow guidance arises from the posterior of the cells. We first attached anti-ICAM-3 labelled micron-sized beads on the uropod of T lymphocytes, where adhesion molecule ICAM-3 is specifically enriched. When exposed to flow, the cells with beads on their uropod migrate upstream similar to normal cells without beads, whereas cells attached in multiplets to a common bead have an orientation clearly independent of flow ( Fig. 3d and Supplementary Movie 5 ). In fact, cell multiplets form quasi-stable patterns with an immobile ‘crosslinking’ point at the centre and cells pulling radially in diverging directions with regular angles between cells. The independence of orientation with flow is consistent with the fact that mutual tractions between cells induced by their powerful motility machinery overcome the hydrodynamic shear stress on each cell [4] . Moreover, according to Newton’s law, the sum of forces on the immobile bead of a multiplet is null at equilibrium, and considering that each cell roughly develops the same force and pulls away from its uropod, multiplets of n cells are expected to form regular star patterns with angles between branches of 2 π/n . The static behaviour of multiplet suggests therefore that it is not directly the flow direction but rather the position of the uropod that is determinant for a cell forward orientation. The dynamic role of uropod on cell's orientation can then be observed with cells escaping unstable positions. In Fig. 3e and Supplementary Movie 6 , the cell-trailing edge is trapped on a surface defect, and cell orientation is opposite to the attachment point, such as in a multiplet. The flow is orientated from right to left in opposition to cell orientation, so that the cell is initially 180° apart from its equilibrated upstream-bound orientation. When the attachment point breaks, the uropod immediately initiates a repositioning downstream of the cell, and the cell resumes a normal upstream crawling within 100 s. Hence, if the hydrodynamic stimulation is insignificant compared with the powerful cell motility machinery and therefore insufficient to directly alter the velocity and orientation of a crawling cell, it easily orients the free-rotating uropod downstream of a cell body, which then manifestly triggers the reorientation of the whole cell. Uropods seemingly act similar to a wind vane that can direct cells direction. Uropod deflection controls steering of cells To challenge the role of uropod as a wind vane-type regulator of cell migration direction, we then quantified the external stimulus required to actuate the guidance mechanism. In a first experiment, we attached large beads of 12 μm diameter to the cells’ uropod to amplify the hydrodynamic drag on the cell rear. Cells equipped with such amplifiers are expected to be more sensitive to surrounding flow conditions. Cell velocity is not dependent on bead presence ( Supplementary Note 2 and Supplementary Fig. 2 ), whereas upstream orientation is indeed systematically more pronounced as compared with control cells ( Fig. 4a ). Considering that the size of the cell rear is dominated by the size of the bead, and that beads under flow are pushed in contact to the surface, the hydrodynamic drag force, F d , on the cell rear can be estimated by the force on a sphere settling on a flat surface and submitted to a flow, F d ≈ 32 a 2 σ , where a is the diameter of the bead and σ is the local shear stress [17] . The onset of orientation versus flow corresponds to a force on the bead of ~30 pN. This range of force is accessible with magnetic actuation of beads. We therefore equipped cells with magnetic beads on their uropod and exposed them to a permanent magnet. As compared with flow experiments, mechanical actuation applies here only on the uropod and not on the whole cell body. In these conditions, cells orient their path in the opposite direction to the magnetic force ( Fig. 4b ). Hence, whether by flow or magnetic actuation, the uropod acts as a steering wheel of the ‘crawling cell’ vehicle. By actuating this steering wheel, one can navigate individual lymphocytes like one would a radio-controlled toy, as shown in the experiment in Fig. 4c and Supplementary Movie 7 . The distance between the cell equipped with a magnetic bead and the tip of a magnetic tweezers is here maintained constant via a dynamic control of the microscopic stage, and sequential applications of hydrodynamic and magnetic forces making an angle of 90° allows one to drive lymphocytes on a step-like pathway. 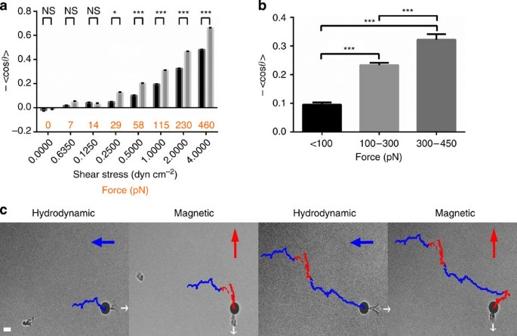Figure 4: Quantification of cell steering by uropod. (a) Index of directionality<cosθ>versus axis of flow direction as a function of shear stress intensity (blackxaxis) for control lymphocytes (black bars) and lymphocytes with 12-μm diameter magnetic beads attached to cells uropods (grey bars). The force on the cell rear,Fr, exerted by the bead is indicated in orange onxaxis17. Data for each condition were calculated for >50 cells after four independent experiments. Error bars indicate±s.e.m. *P<0.05, **P<0.01, ***P<0.001 (two tailed unpairedt-test). (b) Index of directionality<cosθ>versus axis of magnetic gradient as a function of horizontal magnetic force exerted on the beads on the cells uropods.Nsteps>20,000. Data are mean±s.e.m. of three independent experiments. *P<0.05, ***P<0.001 (one way analysis of variance followed by the Tukey multiple-comparison test). (c) Driving a lymphocyte using the uropod as a steering wheel. Sequence of images at timest=720 s,t=1,200 s,t=2,380 s andt=3,000 s, of a single lymphocyte with a 12-μm diameter magnetic bead attached to its uropod and submitted alternatively to hydrodynamic force (blue arrow) pulling the bead to the left and to a magnetic force (red arrow) pulling the bead to the top. The cell is kept immobile in the field of view via a dynamic control of the microscope X-Y stage to maintain the distance between the bead and the magnetic tip constant. Dots indicate the successive relative positions of the cell every 2 s during hydrodynamic (blue dots) and magnetic (red dots) actuation. White arrows indicate cell polarization direction. The trajectory displays steps with blue horizontal segments and red vertical segments corresponding to the cycles of, respectively, hydrodynamic and magnetic actuation of 200 pN with 90° angle. Scale bar, 10 μm. NS, not significant. Figure 4: Quantification of cell steering by uropod. ( a ) Index of directionality <cosθ> versus axis of flow direction as a function of shear stress intensity (black x axis) for control lymphocytes (black bars) and lymphocytes with 12-μm diameter magnetic beads attached to cells uropods (grey bars). The force on the cell rear, F r , exerted by the bead is indicated in orange on x axis [17] . Data for each condition were calculated for >50 cells after four independent experiments. Error bars indicate±s.e.m. * P <0.05, ** P <0.01, *** P <0.001 (two tailed unpaired t -test). ( b ) Index of directionality <cosθ> versus axis of magnetic gradient as a function of horizontal magnetic force exerted on the beads on the cells uropods. N steps >20,000. Data are mean±s.e.m. of three independent experiments. * P <0.05, *** P <0.001 (one way analysis of variance followed by the Tukey multiple-comparison test). ( c ) Driving a lymphocyte using the uropod as a steering wheel. Sequence of images at times t =720 s, t =1,200 s, t =2,380 s and t =3,000 s, of a single lymphocyte with a 12-μm diameter magnetic bead attached to its uropod and submitted alternatively to hydrodynamic force (blue arrow) pulling the bead to the left and to a magnetic force (red arrow) pulling the bead to the top. The cell is kept immobile in the field of view via a dynamic control of the microscope X-Y stage to maintain the distance between the bead and the magnetic tip constant. Dots indicate the successive relative positions of the cell every 2 s during hydrodynamic (blue dots) and magnetic (red dots) actuation. White arrows indicate cell polarization direction. The trajectory displays steps with blue horizontal segments and red vertical segments corresponding to the cycles of, respectively, hydrodynamic and magnetic actuation of 200 pN with 90° angle. Scale bar, 10 μm. NS, not significant. Full size image Upstream crawling works without usual guidance signalling If the uropod wind vane detects flow direction and guides cells, it remains unclear how the transmission of cue detection into a steering command to the whole cell is performed. The existence of a specific internal signalling triggered by cue detection has been tested by visualizing intracellular calcium level changes using BD PBX labelling ( Fig. 5a and Supplementary Movie 8 ). Clearly, interactions between the uropod and flow trigger no change in calcium concentration. Since calcium is involved in many signalling pathways, these data challenge the existence of an active transmission between cue detection and directivity. Furthermore, high-affinity integrins and/or calcium channels have been reported as key element in the active mechanism of neutrophils recruitment and guidance [18] , [19] . However, with effector T lymphocytes, we found that inhibitors of calcium-release-activated channels ( Fig. 3 and Supplementary Note 3 ), as well as promoters of either integrins high- or low-affinity states had a weak effect on crawling speed and direction in the presence and absence of external flow ( Supplementary Fig. 4 and Supplementary Note 4 ). Finally, phosphoinositide 3-kinases played an important role in the active gradient sensing machinery in chemotaxis of amoebae Dictyostelium [20] , [21] , and was also reported to be involved in galvanotaxis of keratocytes [22] and mechanotaxis of Dictyostelium discoideum [23] , Entamoeba histolytica [24] and endothelial cells [25] . However, inhibitors of phosphoinositide 3-kinases or G-protein-coupled receptors ( Supplementary Note 5 and Supplementary Fig. 5 ) hardly affect migration and upstream mechanotaxy of effector T cells. Altogether, these data show that common intracellular guidance signalling pathways involved in various cell guiding mechanisms are not involved in upstream mechanotaxis of effector T lymphocytes. This supports exploration of alternative mechanisms for transmission between cue detection and cell direction. 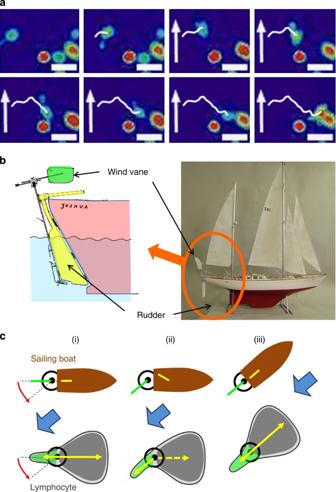Figure 5: Self-steering under passive uropod/wind vane regulation. (a) Flow triggers no internal calcium signalling. Sequence of images taken every 1 min of relative intracellular calcium levels in crawling lymphocytes under flow using fluo-4 PBX. Calcium sensor intensity is displayed with a pseudo-colour glow scale (red, highest to blue, lowest activity). Flow is null in the beginning, and a white arrow indicating flow direction appears when flow is started with a shear stress of 8 dyn cm−2. Calcium level is unaffected by flow application, but strongly increased upon cell encounters (last image). White line indicates the track of the migrating cell of interest. Scale bars 20 μm; sequence is representative of 10 cells after three independent experiments. (b) Wind vane steering regulation on a sailing boat (adapted from ref.26). At the rear of the boat, an immersed rudder (yellow) serves to steer the boat and an wind vane in the air (green) is sensitive to wind direction. The wind vane is coupled to a trim-tab fixed on the rudder. The rotation of the wind vane/trim-tab, which requires little power, is actuated by the wind, whereas the hydrodynamic coupling between trim-tab and rudder (yellow) induces a strong hydrodynamic torque on the rudder and the required power to turn the boat. (c) Comparative self-steering model for a sailing boat and a lymphocyte. (i) A faint external cue, wind or flow (blue arrow), induces a slight rotation of the wind vane or uropod (green), which (ii) biases the powerful steering machinery (yellow) of the boat (rudder) or of the lymphocyte (the front rear axis of polarization). (iii) The boat or cell turns until the wind vane or uropod is aligned with the external flow and the steering mechanism is back to neutral position. Figure 5: Self-steering under passive uropod/wind vane regulation. ( a ) Flow triggers no internal calcium signalling. Sequence of images taken every 1 min of relative intracellular calcium levels in crawling lymphocytes under flow using fluo-4 PBX. Calcium sensor intensity is displayed with a pseudo-colour glow scale (red, highest to blue, lowest activity). Flow is null in the beginning, and a white arrow indicating flow direction appears when flow is started with a shear stress of 8 dyn cm −2 . Calcium level is unaffected by flow application, but strongly increased upon cell encounters (last image). White line indicates the track of the migrating cell of interest. Scale bars 20 μm; sequence is representative of 10 cells after three independent experiments. ( b ) Wind vane steering regulation on a sailing boat (adapted from ref. 26 ). At the rear of the boat, an immersed rudder (yellow) serves to steer the boat and an wind vane in the air (green) is sensitive to wind direction. The wind vane is coupled to a trim-tab fixed on the rudder. The rotation of the wind vane/trim-tab, which requires little power, is actuated by the wind, whereas the hydrodynamic coupling between trim-tab and rudder (yellow) induces a strong hydrodynamic torque on the rudder and the required power to turn the boat. ( c ) Comparative self-steering model for a sailing boat and a lymphocyte. (i) A faint external cue, wind or flow (blue arrow), induces a slight rotation of the wind vane or uropod (green), which (ii) biases the powerful steering machinery (yellow) of the boat (rudder) or of the lymphocyte (the front rear axis of polarization). (iii) The boat or cell turns until the wind vane or uropod is aligned with the external flow and the steering mechanism is back to neutral position. Full size image Cells can navigate under passive wind vane self-steering A maritime analogy allows us to propose a minimal and plausible model of guiding mechanism for lymphocytes, which requires no unknown signalling to transduce cue detection into motility machinery remodelling. Sailors have used passive mechanical wind vane self-steering gears ( Fig. 5b ) to navigate single-handed on sailing boats [26] , [27] , long before the advent of active electronic self-steering systems guided by compass or GPS signals. In the functioning of wind vane self-steering gears, a wind vane is adjusted to face into the wind when the boat is on the right course. When the boat wanders off-course, the wind strikes the wind vane from one side and the slight rotation of the wind vane by the faint wind force biases a steering system (a steering wheel or a trim-tab on the rudder) that has sufficient power to reorient the boat ( Fig. 5c ). Similarly, the uropod of lymphocytes has a wind vane behaviour that is sensitive to faint flows. The change of uropod wind vane orientation biases directly the rear-front axis of cell polarization ( Fig. 5c ), and the robust mechanism of polarization maintenance can then trigger cell steering by re-establishing the lamellipod/uropod alignment. In this view, there is no activation of a specific internal signalling cascade by specialized sensors, such as in chemotaxis. The internal regulation of rear-front polarization may remain unchanged with or without mechanical stimulation by flow, and cells will respond passively to the external solicitation with upstream phenotype. Perturbation of the self-steering system by inhibitors To test further the idea that the uropod/wind vane coupled to the on-going rear-front polarization regulation is the steering mechanism of lymphocytes flow mechanotaxis, we then applied drugs to perturb the main cogs of this machinery, first the transmission system (cell polarity) and then the detection system (cell uropod/wind vane). The uropod contains a microtubule network [11] that is known to participate in maintaining cell cortical polarity [28] . Disruption of microtubules with nocodazole ( Fig. 6a , Supplementary Movie 9 ) or vinblastin provoked frequent turning of cells, and diminished the average orientation of cells with flow ( Fig. 6a,b , Supplementary Note 6,7 and Supplementary Fig. 6 ), consistent with previous observations on neutrophils [29] and lymphocytes [30] . Perturbation of cell polarity by nocodazole is clearly revealed by the much wider shape of the lamellipod that tends to extend in 360° directions ( Fig. 6c and Supplementary Movie 10 ). Within the model of the wind vane-regulated self-steering, impairment of the rear-front polarization, that is, of the transmission system of flow direction detection into steering command, is straightforwardly consistent with the observed loss of guidance with flow. We then treated cells with blebbistatin, a potent inhibitor of actomyosin activity. Blebbistatin-treated cells present a strong elongation of their uropods ( Fig. 6c and Supplementary Movie 11 ), as previously observed [31] , and a marked increase of cell orientation with flow ( Fig. 6b , Supplementary Note 7 and Supplementary Movie 12 ). Adherence with the substrate is not responsible for uropod rearward elongation. The uropods of blebbistatin-treated cells remain markedly non-adherent, as revealed by images of the cells footprint on the substrate ( Supplementary Movie 13 ) and by uropod instantaneous adaptation to changes in flow direction ( Supplementary Movie 14 ). In fact, decrease of actomyosin activity is known to diminish microvilli stability and promote membrane unfolding under stress [32] , which explains the elongation of uropods under flow. Within the model of the wind vane-regulated self-steering, a wind vane of larger size has a higher sensitivity to flow direction, which is consistent with the observed increase of guidance efficiency with flow. More quantitatively, we determined the average uropods length L u for each experimental conditions and then plotted the directionality < cos θ> of cells treatment against σ * L u 2 , which characterizes the strength of the torque to align the uropods ( Fig. 6d ). All data with and without blebbistatin follow a single master curve, which is consistent with the size of the uropod/wind vane being the main cause of guidance sensibility enhancement by blebbistatin treatment. Finally, we found a net correlation between the persistence time in absence of flow, as determined at the transition between the directional and diffusive regime ( Fig. 2b ), and the efficiency of the guidance by flow ( Fig. 6e ). This observation is in accordance with a guidance model relying on the properties of the polarization mechanism that are already in place in absence of flow. 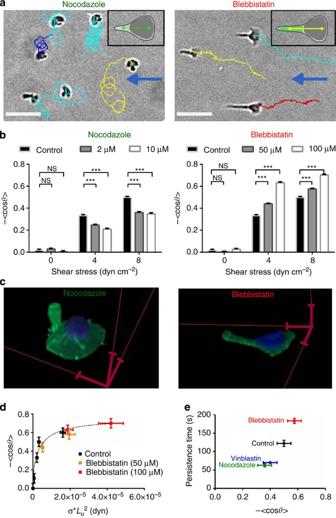Figure 6: Perturbation of the wind vane self-steering system with inhibitors of microtubules and actomyosin contractility. (a) Cells trajectories superposed to transmission image at a shear stress of 8 dyn cm−2, and with nocodazole and blebbistatin at, respectively, 10 and 100 μM. Blue arrows indicate flow direction. Scale bars, 50 μm. Insets inaare mechanistic cartoons of nocodazole- and blebbistatin-treated cells with loose transmission mechanism (dotted green arrow, left) and enlarged detection mechanism (green uropod, right). (b) Index of directionality<cosθ>versus shear stress. For each condition, data are mean±s.e.m of one experiment withNcells> 100, representative ofn=3 experiments. ***P<0.001 (two tailed unpairedt-test). (c) Three-dimensional confocal microscopy images of cells stained for the membrane (green) and the nucleus (blue) in the absence of flow with nocodazole 10 μM (left) and blebbistatin 100 μM (right). Red scale bars, 5 μm. (d) Index of directionality<cosθ>versus shear stress multiplied by the square of the average uropod lengthσ*Lu2of effector T cells for control (black dots), and for blebbistatin treatments 50 μM (orange dots) and 100 μM (red dots). All data follow a single master curve (dotted line). Data are mean±s.e.m of three independent experiments withNcells> 20 per condition. Horizontal errors bars are calculated using s.e.m ofLu. (e) Persistence time of the ballistic regime in the random migration in absence of flow versus the index of directionality<cosθ>in presence of a flow of 8 dyn cm−2for normal cells and for cells with treatment nocodazole 10 μM, blebbistatin 100 μM and vinblastin 10 nM. Data are mean±s.e.m of three independent experiments withNcells> 200 per condition. NS, not significant. Figure 6: Perturbation of the wind vane self-steering system with inhibitors of microtubules and actomyosin contractility. ( a ) Cells trajectories superposed to transmission image at a shear stress of 8 dyn cm −2 , and with nocodazole and blebbistatin at, respectively, 10 and 100 μM. Blue arrows indicate flow direction. Scale bars, 50 μm. Insets in a are mechanistic cartoons of nocodazole- and blebbistatin-treated cells with loose transmission mechanism (dotted green arrow, left) and enlarged detection mechanism (green uropod, right). ( b ) Index of directionality <cosθ> versus shear stress. For each condition, data are mean±s.e.m of one experiment with N cells > 100, representative of n =3 experiments. *** P <0.001 (two tailed unpaired t -test). ( c ) Three-dimensional confocal microscopy images of cells stained for the membrane (green) and the nucleus (blue) in the absence of flow with nocodazole 10 μM (left) and blebbistatin 100 μM (right). Red scale bars, 5 μm. ( d ) Index of directionality <cosθ> versus shear stress multiplied by the square of the average uropod length σ * L u 2 of effector T cells for control (black dots), and for blebbistatin treatments 50 μM (orange dots) and 100 μM (red dots). All data follow a single master curve (dotted line). Data are mean±s.e.m of three independent experiments with N cells > 20 per condition. Horizontal errors bars are calculated using s.e.m of L u . ( e ) Persistence time of the ballistic regime in the random migration in absence of flow versus the index of directionality <cosθ> in presence of a flow of 8 dyn cm −2 for normal cells and for cells with treatment nocodazole 10 μM, blebbistatin 100 μM and vinblastin 10 nM. Data are mean±s.e.m of three independent experiments with N cells > 200 per condition. NS, not significant. Full size image In the end, whereas chemotaxis is based on an active self-steering system (such as electronic navigation device), with an external cue detected and specifically processed to activate guidance signalling and new functions at different locations in the cell, flow mechanotaxis can be explained by a passive self-steering system (such as mechanical wind vane device), with only continually maintained polarity signalling and without new internal signalling specific to the external cue. This scenario is also consistent with the fact that active chemotaxis allows adaptation to increasing signals as cells travel up a gradient on four orders of magnitude [6] , whereas passive flow mechanotaxis is only efficient for a limited range of stimuli. The physiological benefit of flow orientation is currently unknown for lymphocytes and more generally for neutrophils [16] , endothelial cells [9] or amoebae [23] . The fact that neutrophils crawl downstream [16] and T lymphocytes upstream [4] while migrating on the same adhesive ligand, challenges the idea of a universal flow-guided mechanism selected to favour extravasation. Furthermore, as upstream crawling may not rely on a specific signalling mechanism, one cannot exclude that flow orientation may be a fortuitous consequence of uropod morphology. Nevertheless, the robust flow mechanotaxis behaviour of T lymphocytes supports the idea of a mechanism purposely selected by evolution. If evolution is not requisite to shape a passive mechanism, it may nevertheless play a direct role, for instance, by tuning the morphology of the uropod that is the trigger of the mechanism. We may speculate that the evolutionary advantage of upstream crawling could be to guide lymphocytes towards the epicentre of signalling endothelial zone, if their arrest occurred downstream of the epicentre. Flow devices Devices to change flow direction by 90° were fabricated using standard soft lithography routines [13] . A positive mould was created with SU-8 2100-negative resins (Microchem, USA) on silicon wafers (Siltronix, France), then replicas were moulded in polydimethylsiloxane (PDMS) elastomer (Sylgard 184, Dow Corning, USA) and sealed on glass coverslides via plasma activation (Harricks Plasma, USA). Ports to plug inlet and outlet reservoirs were punched with a 1-mm outer diameter needle. The device is composed of two entries leading to perpendicular channels and one output. Switching injection from one entry to the other induces a change of flow direction by 90° in the confluence region between the channels connected to the entries. Devices for experiments using magnetic actuation were made of two glass coverslides separated by a 300-μm-thick PDMS film and sealed by plasma activation. The channel (3 × 45 mm) was cut in a 300-μm-thick PDMS film from Sterne (Cavaillon, France) using a cutting plotter from Graphtec (Yokohama, Japan). 1-mm diameter holes for entry of fluid in the upper glass coverslide were drilled by sandblasting. A thin upper face was chosen to minimize the distance between the magnetic tweezers tip and the beads in the liquid cell in order to maximize the accessible magnetic actuation force. Flow devices were coated overnight at 4 °C with 10 μg ml −1 human ICAM-1-Fc (R&D Systems, Minneapolis, MN, USA) in PBS (Gibco, Carlsbad, CA, USA). Channels were subsequently blocked with 2.5% bovine serum album (BSA) (Axday, Dardilly, France) and 2.5% Pluronic F-108 (BASF, Ludwigshafen, Germany) in PBS (Gibco, Life Technologies Corp., Grand Island, NY, USA) for 30 min at room temperature. Channels were rinsed with PBS. Cells were then added in complete culture medium, allowed to equilibrate for 10 min and then rinsed with medium. Flow control In the device to change flow direction by 90°, flow rates were controlled via a difference of levels between two fluid reservoirs connected to the inputs and output of the device. An automatic multiways valve (Nonapeak, Scivex, Oak Harbour, WA, USA) was inserted between the entry reservoir and the two entries to restrict connection of a single entry at a time to the entry reservoir. Switching the valve from one entry to the other allowed a change of the flow direction in the device in a fraction of second. For all experiment in straight channels on cells with beads attached to their uropod, the flow was controlled using two syringe pumps (Nemesys, Cetoni GmbH, Germany) and two two-way automatic valves assembled in a closed circuit to provide a continuous and unidirectional flow in the channels upon filling/emptying cycles of each syringe. Microscopic observations We used a Zeiss Observer Z1 microscope (Carl Zeiss, Oberkachen, Germany) piloted with μManager [14] and MATLAB (The MathWorks Inc, Natick, MA, USA). The microscope was equipped with a CoolSnap HQ CCD camera (Photometrics, Tucson, AZ, USA) and different Zeiss objectives for bright-field and differential interferential contrast (DIC) mode (Plan-Apochromat × 10/0.3, × 20/0.8 and × 63/1.4) for RICM mode (Neofluar 63/1.25 antiflex) and for TIRF mode ( × 100/1.45). The source was an X-cite 120Q lamp (Exfo, Mississauga, Canada) for bright-field, differential interferential contrast and RICM mode and a laser for TIRF. A narrow band-pass filter ( λ =546 nm±12 nm) was used for RICM, whereas the wavelength was of 488 nm for TIRF. Confocal microscopy was performed on a Leica SP5 confocal equipped with LAS AF Lite Software. Cells and reagents Whole blood from healthy adult donors was obtained from the ‘Etablissement Francais du Sang’. Peripheral blood mononuclear cells were recovered from the interface of a Ficoll-Paque PLUS (GE Healthcare, Pittsburgh, PA, USA) gradient. The peripheral blood mononuclear cells were then stimulated for 72 h with 10 mg ml −1 phytohemagglutinin- L (Roche Diagnostics, Indianapolis, IN, USA) at 37 °C/5% CO 2 and subsequently cultivated in Roswell Park Memorial Institute Medium (RPMI) 1640 supplemented with 25 mM HEPES and 25 mM GlutaMax (Gibco), 10% fetal calf serum (Lonza, Basel, Switzerland) in the presence of interleukin-2 (50 ng ml −1 ; Miltenyi Biotec, Auburn, CA, USA). Cells were typically used 7–10 days after stimulation. At the time of use, the cells were >95% positive for pan-T lymphocyte marker CD3ε and negative for T lymphocyte activation marker CD69 as judged by flow cytometry. Pan-LFA-1 antibody mAb38 was a generous gift of N. Hogg (UK Cancer Research, UK). Alexa 488-labelled goat anti-mouse secondary antibody and fluorescein isothiocyanate-labelled wheat germ agglutinin was obtained from Life Technologies (Carlsbad, CA, USA). Biotionylated anti-ICAM3 was obtained from Abcam (Cambridge, UK). Hoechst 33342, vinblastin and nocodazole was obtained from Sigma-Aldrich (St Louis, MO USA), wortmannin from Calbiochem (SanDiego, CA, USA), blebbistatin from Fisher Bioblock Scientific (Illkirch, France) and fluo-4 PBX Calcium Assay Kit from BD Biosciences (San Jose, CA, USA). Cell treatments For fluorescence staining of cells in confocal and TIRF microscopy, cells were allowed to adhere to ICAM-1-Fc-coated microfluidic channels for 20 min at 37 °C before fixation with 3.5% paraformaldehyde. Samples were subsequently labelled with Wheat Germ Agglutinin, mAb38 and/or Hoechst 33342 as per manufacturer’s instructions, and stabilized with ProLong Gold (Life Science Technologies). For experiments with nocodazole and blebbistatin, stock solutions were prepared in DMSO following manufacturer’s specification and stored at −20 °C, and then diluted in culture medium for flow experiments with a DMSO content<0.5%. Cells were injected in microfluidic channels with culture medium and let settled for 5 min to allow adhesion. Drug solutions were then injected at low shear stress (<1 dyn cm −2 ) and after a 10-min incubation period, experiments under flow were started keeping the same concentration condition in the flowing fluid. For calcium imaging experiments, cells were first injected in a microfluidic channel with culture medium and were allowed to settle for 5 min to allow adhesion, then a BD PBX solution (according to manufacturer’s instruction) diluted to 2,000 × (~0.5 μM) was injected for 30 min at 37 °C in the dark. Cells were finally washed with RPMI medium supplemented with 2% fetal calf serum and 10 mM HEPES. Cell tracking and data analysis A home-made programme was developed with MATLAB software (The MathWorks, Natick, MA, USA) to track migrating cells and analyse their pathway properties [15] . In order to get an indication of the amount of movement in a particular direction, we computed the average cosine of the angle, < cos θ> , between this direction and the orientation of the cell path for two positions separated by 50 s. This index is equivalent to the chemotactic index that is usually used to quantify the migration direction relative to gradients of chemotactic factors. The average speed of a cell is calculated as the ratio between the contour length of the total trajectory and the corresponding time of migration. Magnetic actuation Magnetic fields were applied with a permanent magnet lying directly on top of the straight channel flow device or with a custom-made magnetic tweezers setup positioned in the close vicinity of the flowing channel. We used two types of magnetic beads with diameter 2.8 μm (Dynabeads M-270 Streptavidin, Invitrogen, Norway) and 12 μm (micromod, M-Streptavidin 08-19-124). To equip cells uropods with magnetic beads, 10 μl of streptavidin beads stock solution were washed three times in 100 μl PBS solution, and 2 μl of biotinylated anti-ICAM3 antibody was added for 30 min. Beads were then washed three times in PBS solution and finally re-suspended in 100 μl of culture medium. Cells were injected in the flow devices in complete culture medium and were allowed to equilibrate for 10 min at 37 °C before rinsing. The solutions of antibody-coated beads were then injected and allowed to equilibrate with crawling cells for roughly 15 min. The beads lying on the lower surface were progressively picked up by crawling cells upon random encounters. When an appropriate number of crawling had picked up a bead and before too many cells had picked up multiple beads, channels were rinsed, which eliminated unattached beads. Samples were imaged with an inverted microscope, whereas the magnetic field source (magnet or tweezers) were positioned above the sample. Flow devices were turned upside-down to minimize the distance between the cells and the magnetic field source ( Supplementary Fig. 8 ), the lowest limit being imposed by the channel ceiling made by a microscope slide of thickness 130 μm. With magnetic tweezers, the tip was placed at 220 μm from the magnetic bead attached to a cell, and the distance was kept constant during the experiment by maintaining the bead in the centre of the field. The movement of the beads owing to the migration of the carrying cell were dynamically compensated by opposite movement of microscope X-Y stage via an automatic regulation code written in MATLAB and run using μManager interface [14] . Movements of the stage were used to reconstruct the migration trajectory of the cell. Calibration of forces on the beads was performed by measuring the velocity of beads in bulk suspension of known viscosity at different positions in the device. For 12 μm diameter beads, the force applied with the magnetic tweezers was of 120±50 pN, the dispersion being due to the dispersion in diameter and magnetic susceptibility of the beads. How to cite this article: Valignat, M.-P. et al. Lymphocytes can self-steer passively with wind vane uropods. Nat. Commun. 5:5213 doi: 10.1038/ncomms6213 (2014).